Interaction between p68 RNA helicase and Ca2+-calmodulin promotes cell migration and metastasis p68 RNA helicase is a prototypical RNA helicase. Here we present evidence to show that, by interacting with Ca-calmodulin, p68 has a role in cancer metastasis and cell migration. A peptide fragment that spans the IQ motif of p68 strongly inhibits cancer metastasis in two different animal models. The peptide interrupts p68 and Ca-calmodulin interaction and inhibits cell migration. Our results demonstrate that the p68–Ca-calmodulin interaction is essential for the formation of lamellipodia and filopodia in migrating cells. p68 interacts with microtubules in the presence of Ca-calmodulin. Our experiments show that interaction with microtubules stimulates p68 ATPase activity. Further, microtubule gliding assays demonstrate that p68, in the presence of Ca-calmodulin, can function as a microtubule motor. This motor activity may allow p68 to transport Ca-calmodulin to the leading edge of migrating cells. Migration is an essential characteristic of cells in numerous fundamental biological processes [1] , [2] , [3] , [4] , [5] , [6] , including cancer metastasis [7] . Targeting cell migration is a very important strategy for metastasis intervention [8] , [9] . Cell migration is accomplished by a series of highly organized cyclic processes. First, the cells polarize and extend protrusions towards the direction of stimuli. The polarization is led by lamellipodia and filopodia [10] . Accompanying the protrusion, an extensive rearrangement of cell adhesions to the extracellular matrix (ECM) stabilizes the protrusion and functions as an anchor for traction [10] , [11] . Following protrusion, the cell adhesion at the rear side detaches from the ECM [12] . It is believed that formation of the leading edge is driven by cytoskeleton polymerization [13] , [14] , [15] . Many proteins have a role in regulating cytoskeletal rearrangement during migration [16] . Another important feature in the cell migration is that many molecules that have critical role(s) in migration redistribute to the migration leading edge [17] , [18] . Transportation along microtubules (MTs) by families of MT motors is the main mechanism by which proteins and organelles translocate towards the direction of migration [19] , [20] , [21] , [22] . Ca-calmodulin (CaM) is a calcium trigger protein with four EF-hands. The protein activates a wide range of cellular targets to regulate multiple processes in response to Ca 2+ signals [23] . One important molecular mechanism that contributes to the capability of CaM in regulating many cellular processes is its rapid redistribution to subcellular compartments in response to various signals [24] , [25] . CaM is a major factor in connecting Ca 2+ signalling to cell motility in many cell types [26] , [27] . Migration signals trigger spatiotemporal redistribution of CaM to the leading edge of the migrating cell, which is essential for cell motility [28] , [29] , [30] . Although, redistribution of CaM has long been recognized as a mechanism that regulates complex cellular Ca 2+ signals, little is known about how redistribution of CaM is accomplished and its role in cancer metastasis. Here we report that interaction of p68 RNA helicase with CaM is essential for cell migration. Disruption of p68–CaM interaction inhibits cell migration. Interruption of p68–CaM interaction also strongly inhibits cancer metastasis. Our experiments showed that p68, upon interacting with CaM, can act as a MT motor to transport CaM to the leading edge of migrating cells. A peptide fragment of p68 inhibits cancer metastasis We previously reported that phosphorylation of p68 at Y593 mediated the effects of platelet-derived growth factor in promoting epithelial–mesenchymal transition (EMT) by facilitating β-catenin nuclear localization [31] . We asked whether a peptide that spans the nearby region of Y593 with the phosphorylation would be able to inhibit EMT, and could therefore potentially be used for metastasis intervention. To test this, three peptides were synthesized: two peptides span the region of aa 584 to 602 with/without Y593 phosphorylation (referred (ref) to as PepY593 and PepPhoY593 respectively), and a peptide spans the region of aa 549–568 (containing an IQ-like motif, therefore ref to as PepIQ). Both the PepIQ and PepY593 were used as control peptides. Three peptides were fused with the TAT cell permeable sequence at the N-terminus ( Fig. 1a ). The peptides were used to treat mouse xenografts of SW620 cells. We used SW620 because our previous studies revealed high p68 Y593 phosphorylation in these cells [32] , [33] . Xenografts of SW620 metastasize to the lymph nodes, and their metastasis can be analysed by examination of SW620 cells in the spleen [34] . The PepPhoY593 peptide had small effects on SW620 tumour metastasis, whereas cancer metastasis was significantly reduced by the PepIQ peptide ( Fig. 1b ). Tumour growth rates were not affected by treatment with any of the peptides as demonstrated by the anti-Ki-67 immunostaining ( Fig. 1d–f ). Consistent with this, the peptides had no effects on SW620 cell proliferation in vitro ( Fig. 1g ). We also examined whether the peptides would abolish platelet-derived growth factor-stimulated EMT by analysing the EMT markers E-cadherin and vimentin. In consistent with our previous report [31] , the peptide PepPhoY593 treatment led to a decrease in vimentin and an increase in E-cadherin. However, the levels of E-cadherin and vimentin were not affected by the PepIQ and PepY593 ( Supplementary Fig. S1a ). The results suggested that, contrary to our original expectations, the PepPhoY593 had very small effects on cancer metastasis, whereas the PepIQ inhibited metastasis and the inhibitory effect was not due to inhibition of cell proliferation and EMT. The effect of the PepIQ on cancer metastasis was confirmed by an additional treatment using the PepIQ and a control peptide with a scrambled sequence (PepScram) ( Supplementary Fig. S1b–d ). We further verified the effects of the IQ-like sequence on inhibiting cancer metastasis by expression of an enhanced green fluorescent protein (eGFP) fusion protein with the aa 549–568 sequence fused to the C-terminal of eGFP (ref to as GFP-IQ) in SW620 cells ( Supplementary Fig. S2a ). Expression of the GFP-IQ greatly reduced metastasis of the SW620 xenograft, whereas this reduction was not observed with expression of eGFP and vector alone ( Supplementary Fig. S2b–d ). The reduction of cancer metastasis was not due to changes in tumour growth upon expression of the fusion proteins ( Supplementary Fig. S2e ). 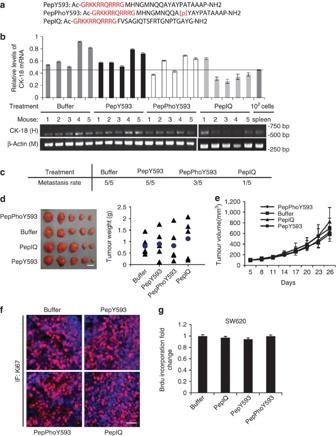Figure 1: The effects of designed peptides on metastasis of xenograft of SW620 tumours. (a) Sequences of three different peptides used in our study. (b) The mRNA levels of human cytokeratin-18 (CK-18) in the spleen extracts of tumour-bearing mice that were treated by different peptides (indicated) 1.5 mg kg−1i.p. were analysed by quantitative RT–PCR (upper) or end point RT–PCR (bottom). The numbers represent individual mouse in each treatment group. The CK-18 mRNA levels were presented as relative levels of CK-18 mRNA by define the level of β-actin mRNA in the same mouse as 1. The mRNA levels of mouse β-actin in the spleen extracts are loading controls. The levels of the CK-18 mRNA in the extracts prepared from the harvested spleen (without tumour implantation) with direct injection of 100 SW620 cells were used as a reference (102cells per spleen). (c) Metastatsis rates of the SW620 xenograft tumours in each treatment group. Tumour metastasis was judged by the CK-18 mRNA levels in the qRT–PCR using that of the 102cells per spleen as the cutoff value. (d) Pictures (left) and weight (right) of harvested SW620 tumours after 28 days growth with 14 days treatment using the indicated peptides. TheP-values between ‘buffer’ and ‘pepIQ’ (P=0.46658) are calculated using pairwise Student’st-test. (e) Tumour growth was monitored by measuring tumour volumes every three days and the tumour volumes were calculated by formula; tumour volume=π/6 × (width) 2 × length. (f) Representative tissue sections were prepared from the harvested tumours and immune fluorescence stained with antibodies against Ki67 (IF: Ki67, red). The blue is 4′,6-diamidino-2-phenylindole stain of cell nucleus. (g) Cell proliferation of SW620 cells that were treated by indicated peptides were measured using a commercial 5-bromodeoxyuridine (BrdU) cell proliferation kit. The proliferation rates are presented as fold changes of BrdU incorporation of the same cultured cells before and after 48 h culturing by defining the initial BrdU incorporation measurement as 1. Scale bars, 1 cm (ford) and 100 μm (forf). Figure 1: The effects of designed peptides on metastasis of xenograft of SW620 tumours. ( a ) Sequences of three different peptides used in our study. ( b ) The mRNA levels of human cytokeratin-18 (CK-18) in the spleen extracts of tumour-bearing mice that were treated by different peptides (indicated) 1.5 mg kg −1 i.p. were analysed by quantitative RT–PCR (upper) or end point RT–PCR (bottom). The numbers represent individual mouse in each treatment group. The CK-18 mRNA levels were presented as relative levels of CK-18 mRNA by define the level of β-actin mRNA in the same mouse as 1. The mRNA levels of mouse β-actin in the spleen extracts are loading controls. The levels of the CK-18 mRNA in the extracts prepared from the harvested spleen (without tumour implantation) with direct injection of 100 SW620 cells were used as a reference (10 2 cells per spleen). ( c ) Metastatsis rates of the SW620 xenograft tumours in each treatment group. Tumour metastasis was judged by the CK-18 mRNA levels in the qRT–PCR using that of the 10 2 cells per spleen as the cutoff value. ( d ) Pictures (left) and weight (right) of harvested SW620 tumours after 28 days growth with 14 days treatment using the indicated peptides. The P -values between ‘buffer’ and ‘pepIQ’ ( P =0.46658) are calculated using pairwise Student’s t -test. ( e ) Tumour growth was monitored by measuring tumour volumes every three days and the tumour volumes were calculated by formula; tumour volume= π /6 × (width) 2 × length. ( f ) Representative tissue sections were prepared from the harvested tumours and immune fluorescence stained with antibodies against Ki67 (IF: Ki67, red). The blue is 4′,6-diamidino-2-phenylindole stain of cell nucleus. ( g ) Cell proliferation of SW620 cells that were treated by indicated peptides were measured using a commercial 5-bromodeoxyuridine (BrdU) cell proliferation kit. The proliferation rates are presented as fold changes of BrdU incorporation of the same cultured cells before and after 48 h culturing by defining the initial BrdU incorporation measurement as 1. Scale bars, 1 cm (for d ) and 100 μm (for f ). Full size image PepIQ abrogates p68–CaM interaction and cell migration How does PepIQ substantially reduce cancer metastasis? Our preceding experiments showed that the peptide had no effects on expression of EMT markers, tumour growth or cell proliferation. It is well known that cell migration is vitally important for cancer metastasis [35] . Thus, cell migration may be the target of the PepIQ peptide. We performed cell migration assays with the SW480 cell line, which is derived from the same cancer patient from whom the SW620 line was derived. SW480 cells have similar migration properties with lower proliferation rates compared with SW620. Clearly, cell migration was almost completely inhibited by PepIQ ( Fig. 2a ). The observed cell migration effects were not due to effects of peptides on cell proliferation ( Supplementary Fig. S2f ). Similarly, cell migration was also dramatically inhibited by stable expression of the GFP-IQ in SW480 cells ( Supplementary Fig. S2g,h ). We then questioned why PepIQ and expression of the GFP-IQ were so effective in inhibiting cell migration. It was demonstrated that p68 interacts with CaM in a number of in vitro binding studies and the IQ-like motif harbours a p68–CaM interaction site [36] , [37] . Thus, it is possible that PepIQ and GFP-IQ competed with p68 to interact with CaM therefore inhibiting cell migration. Thus, we sought to test whether PepIQ interrupts the p68–CaM interaction and consequently inhibits cell migration. We first probed the p68–CaM interaction by coprecipitation with extracts of SW480 cells using CaM beads. Clearly, p68 was precipitated from the extracts by the CaM beads, and the interaction was Ca 2+ dependent ( Fig. 2c ). 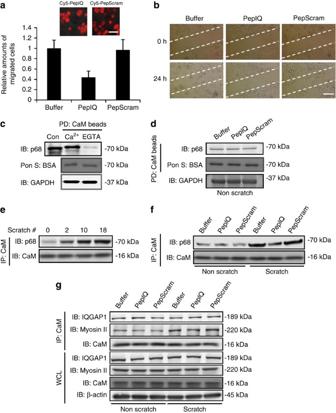Figure 2: Cell migration and p68–calmodulin interactions. Cell migration of SW480 cells was analysed by Boyden chamber assay (a) and monolayer scratch-wound assay (b). Cells were treated by the indicated peptides (10 μg ml−1). The upper two panels inaare representative confocal images of SW480 cells that were treated by the indicated Cy5.5-conjugated peptides, indicating peptide uptake. (a) The number of cells migrating to the lower chamber is presented relative to the number of migrating cells that were treated by buffer. (c) Interaction of p68 with CaM in the presence of 2 mM CaCl2(Ca2+) and 5 mM EGTA (EGTA) was probed by CaM pull-down (PD:CaM beads) followed by immunoblot using antibody against p68 (IB:p68). Cons are the control immunoblot of the cellular extracts using indicated antibody without CaM beads pull-down. (d) Interaction of p68 with CaM in extracts of SW480 cells was probed by CaM pull-down (PD:CaM beads) followed by immunoblot using antibody against p68 (IB:p68). The cells were treated by indicated peptides. Immunoblot of GAPDH (IB:GAPDH) is a loading control. (e) p68 and CaM interaction in extracts prepared from SW480 cells that were subjected to multiple scratch-wound treatment (number of scratches was indicated) analysed by immunoprecipitation of CaM (IP:CaM). (f) p68 and CaM interaction in extracts prepared from SW480 cells that were subjected to 18 scratch-wounds (scratch) or no scratch-wound (non scratch), analysed by immunoprecipitation of CaM (IP:CaM). Cells were treated by the indicated peptides. (g) CaM-IQGAP1 and CaM-Myosin II interactions in extracts prepared from SW480 cells that were subjected to 18 scratch-wounds (scratch) or no scratch-wound (non scratch), analysed by immunoprecipitation of CaM (IP:CaM). The cells were treated by the indicated peptides. Immunoblots of IQGAP1 (IB:IQGAP1), Myosin (IB:Myosin II), and CaM (IB:CaM) in the whole-cell lysate (WCL) indicate the cellular levels of these three proteins. Immunoblot of β-actin (IB:β-actin) in WCL is a loading control. Scale bars, 20 μm (fora) and 100 μm (forb). Figure 2: Cell migration and p68–calmodulin interactions. Cell migration of SW480 cells was analysed by Boyden chamber assay ( a ) and monolayer scratch-wound assay ( b ). Cells were treated by the indicated peptides (10 μg ml −1 ). The upper two panels in a are representative confocal images of SW480 cells that were treated by the indicated Cy5.5-conjugated peptides, indicating peptide uptake. ( a ) The number of cells migrating to the lower chamber is presented relative to the number of migrating cells that were treated by buffer. ( c ) Interaction of p68 with CaM in the presence of 2 mM CaCl 2 (Ca 2+ ) and 5 mM EGTA (EGTA) was probed by CaM pull-down (PD:CaM beads) followed by immunoblot using antibody against p68 (IB:p68). Cons are the control immunoblot of the cellular extracts using indicated antibody without CaM beads pull-down. ( d ) Interaction of p68 with CaM in extracts of SW480 cells was probed by CaM pull-down (PD:CaM beads) followed by immunoblot using antibody against p68 (IB:p68). The cells were treated by indicated peptides. Immunoblot of GAPDH (IB:GAPDH) is a loading control. ( e ) p68 and CaM interaction in extracts prepared from SW480 cells that were subjected to multiple scratch-wound treatment (number of scratches was indicated) analysed by immunoprecipitation of CaM (IP:CaM). ( f ) p68 and CaM interaction in extracts prepared from SW480 cells that were subjected to 18 scratch-wounds (scratch) or no scratch-wound (non scratch), analysed by immunoprecipitation of CaM (IP:CaM). Cells were treated by the indicated peptides. ( g ) CaM-IQGAP1 and CaM-Myosin II interactions in extracts prepared from SW480 cells that were subjected to 18 scratch-wounds (scratch) or no scratch-wound (non scratch), analysed by immunoprecipitation of CaM (IP:CaM). The cells were treated by the indicated peptides. Immunoblots of IQGAP1 (IB:IQGAP1), Myosin (IB:Myosin II), and CaM (IB:CaM) in the whole-cell lysate (WCL) indicate the cellular levels of these three proteins. Immunoblot of β-actin (IB:β-actin) in WCL is a loading control. Scale bars, 20 μm (for a ) and 100 μm (for b ). Full size image We then probed whether PepIQ affected the p68–CaM interaction by the same CaM beads pull-down assay. Clearly, the peptide treatment did not lead to dramatic changes in the p68–CaM interaction ( Fig. 2d ). As we observed that PepIQ greatly inhibited cell migration, we reasoned that the peptide might interfere with the p68–CaM interaction under conditions of migration stimulation, and the p68–CaM interaction itself could also be affected by migration induction. Thus, we examined the p68–CaM interaction in response to migration stimuli by coimmunoprecipitation with extracts of SW480 cells using an antibody against CaM. To induce migration, we used scratch-wounds on the culture plate. A strong increase in p68 and CaM coimmunoprecipitation was observed in the SW480 cells that were subjected to multiple scratch-wounds, and the extent of increase was dependent upon the number of scratches introduced ( Fig. 2e ). Similarly, there was a strong increase in p68 and CaM coprecipitation upon EGF treatment ( Supplementary Fig. S3a,b ). Measurement of the changes in cell migration revealed a close correlation between the increase in the p68–CaM interaction and cell migration under EGF treatment ( Supplementary Fig. S3c ). The results suggest that cell migration strengthened the p68–CaM interaction. As the IQ-like motif harbours the site for the Ca 2+ -dependent p68–CaM interaction [38] , we asked whether the increase in the p68–CaM interaction induced by cell migration requires the IQ-like motif, and used a mutant that carries mutations IQ to MA (ref to as IQ-M). HA-IQ-M was exogenously expressed in SW480 cells in which endogenous p68 was knocked down. HA-IQ-M coprecipitated with CaM. However, the scratch-wound-dependent enhancement in p68–CaM interaction was not observed with the IQ-M mutant ( Supplementary Fig. S3d ). To test whether PepIQ abolished the enhancement of the p68–CaM interaction induced by cell migration, we probed the p68–CaM interaction in cell lysates of SW480 cells that were treated by the peptide. It was clear that the strong increase in the p68–CaM interaction upon multiple scratches was not observed with cells that were treated by the peptide ( Fig. 2f ). Similarly, the p68–CaM interaction was not dramatically strengthened upon migration stimuli in SW480 cells in which GFP-IQ was expressed. Coprecipitation of CaM and GFP-IQ was detected from extracts of the scratch-wound cells ( Supplementary Fig. S3e ), indicating that GFP-IQ competed with p68 for CaM interaction. Many proteins interact with CaM by their IQ motifs [39] , [40] . Examples of the IQ motif containing proteins that interact with CaM are IQGAP1 and Myosin-II. It is well known that IQGAP1 and Myosin-II, and their interaction with CaM, are important for cell migration [41] , [42] , [43] . To test whether PepIQ disrupted the interaction of IQGAP1 or Myosin-II with CaM, we carried out the coimmunoprecipitation with cell extracts of SW480 cells that were treated by PepIQ with/without multiple scratches, using the antibody against CaM. Immunoblots of the coprecipitates indicated that the IQGAP1–CaM and Myosin–CaM interactions were not affected by the PepIQ treatment regardless whether the cells were treated or not by the scratch-wound ( Fig. 2g ). The results indicate that PepIQ likely disrupts the p68 and CaM interaction specifically. The results also excluded a possibility that PepIQ sequestered all CaM in the cells therefore inhibiting cell migration. Thus, our experiments supported the notion that the cell migration strengthened the p68–CaM interaction, and that PepIQ disrupted the p68–CaM interaction induced by migration thus inhibiting cell migration. On the basis of preceding experiments, we predicted that the p68–CaM interaction would be critical for cell migration. The hypothesis was tested by both Boyden chamber and scratch-wound assays. Endogenous p68 was knocked down in SW480 cells and HA-p68s, wild-type (WT), IQ-M, LGLD (an ATPase activity deficiency mutant [44] ), or Y593F [31] , was expressed in the cells ( Fig. 3a ). Boyden chamber assays showed that knockdown of p68 results in a dramatic reduction in cell migration, which could be fully recovered by expression of WT p68, but not by the IQ-M mutant. As a control, cell migration could also be rescued by expression of a mutant that carries a mutation at an irrelevant site (Y595F) ( Fig. 3b ). Interestingly, expression of an ATPase-deficient mutant LGLD did not rescue cell migration ( Fig. 3b ), indicating that the ATPase activity of p68 is required for cell migration. We further confirmed the role of the p68–CaM interaction in cell migration by scratch-wound assays ( Fig. 3c ). Immunofluorecence staining using anti-HA antibody revealed that no HA-IQ-M- and HA-LGLD-expressing cells migrated to the wounds, whereas p68 WT-expressing cells migrated to the wound areas normally ( Fig. 3d ). These experiments showed that the p68–CaM interaction is required for cell migration. 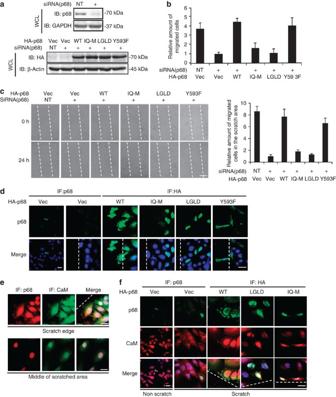Figure 3: p68 and CaM interaction is essential for cell migration and for CaM localization. (a, upper) Levels of p68 in the p68 knockdown SW480 cells were examined by immunoblot in whole-cell lysates (WCLs). (a, bottom) Levels of exogenously expressed HA-p68s, WT and indicated mutants, were analysed by immunoblots of WCLs using anti-HA antibody. Immunoblots of GAPDH and β-actin are loading controls. (b) Migration of SW480 cells in which endogenous p68 was knocked down by RNAi and HA-p68s, WT and mutants (indicated), were exogenously expressed, was analysed by Boyden chamber assays. The number of cells migrating to the lower chamber was measured relative to the number of migrating cells in which the empty vector was transfected. (c, left panel) Migration of SW480 cells in which endogenous p68 was knocked down by RNAi and HA-p68s, WT and mutants (indicated) were exogenously expressed, revealed by phase contrast microscopy 0 and 24 h after scratch-wounds were introduced into the cell culture plates. (a, right panel) Quantification of the cells in a fixed area that migrated to the scratch area. (d) Representative images of SW480 cells in which endogenous p68 was knocked down by RNAi and HA-p68s, WT and mutants were exogenously expressed. HA-p68s was immunostained using anti-HA antibody (green). Endogenous p68 was stained with the antibody p68-RGG (green). 4′,6-Diamidino-2-phenylindole (blue). (e) Representative images of immunofluorescence staining of p68 (red) and CaM (green) in SW480 cells. The cells were treated by scratch-wounding. Upper panel shows cells that located to the scratch edges, bottom panel shows the middle of scratched areas. (f) Representative images of immunofluorescence staining of p68 (green) or exogenously expressed HA-p68s (green), WT or mutants (indicated), and CaM (red) in SW480 cells. The endogenous p68 was knocked down by RNAi. The cells were treated by a scratch-wound (scratch) or no scratch-wound (no scratch) in the culture plate. Error bars inbandcare standard deviations of three independent measurements. Vec is the cells transfected with the empty vector. NT represents the cells treated with non-target RNAi. Scale bars, 100 μm (forc) and 20 μm (ford,eandf). Figure 3: p68 and CaM interaction is essential for cell migration and for CaM localization. ( a , upper) Levels of p68 in the p68 knockdown SW480 cells were examined by immunoblot in whole-cell lysates (WCLs). ( a , bottom) Levels of exogenously expressed HA-p68s, WT and indicated mutants, were analysed by immunoblots of WCLs using anti-HA antibody. Immunoblots of GAPDH and β-actin are loading controls. ( b ) Migration of SW480 cells in which endogenous p68 was knocked down by RNAi and HA-p68s, WT and mutants (indicated), were exogenously expressed, was analysed by Boyden chamber assays. The number of cells migrating to the lower chamber was measured relative to the number of migrating cells in which the empty vector was transfected. ( c , left panel) Migration of SW480 cells in which endogenous p68 was knocked down by RNAi and HA-p68s, WT and mutants (indicated) were exogenously expressed, revealed by phase contrast microscopy 0 and 24 h after scratch-wounds were introduced into the cell culture plates. ( a , right panel) Quantification of the cells in a fixed area that migrated to the scratch area. ( d ) Representative images of SW480 cells in which endogenous p68 was knocked down by RNAi and HA-p68s, WT and mutants were exogenously expressed. HA-p68s was immunostained using anti-HA antibody (green). Endogenous p68 was stained with the antibody p68-RGG (green). 4′,6-Diamidino-2-phenylindole (blue). ( e ) Representative images of immunofluorescence staining of p68 (red) and CaM (green) in SW480 cells. The cells were treated by scratch-wounding. Upper panel shows cells that located to the scratch edges, bottom panel shows the middle of scratched areas. ( f ) Representative images of immunofluorescence staining of p68 (green) or exogenously expressed HA-p68s (green), WT or mutants (indicated), and CaM (red) in SW480 cells. The endogenous p68 was knocked down by RNAi. The cells were treated by a scratch-wound (scratch) or no scratch-wound (no scratch) in the culture plate. Error bars in b and c are standard deviations of three independent measurements. Vec is the cells transfected with the empty vector. NT represents the cells treated with non-target RNAi. Scale bars, 100 μm (for c ) and 20 μm (for d , e and f ). Full size image p68 and CaM interaction affect the localization of CaM and p68 In the immunostaining, we noted two interesting phenomena. (1) We observed a strong cytoplasmic p68 staining only in the migrating cells. When the cells reached their destination, p68 relocalized exclusively back to the cell nucleus ( Fig. 3e ). (2) There were very high levels of p68 staining in the cytoplasm and at the leading edge of the migrating cells, and this staining pattern was not observed in the non-migrating cells ( Fig. 3d ). As p68 interacted with CaM in migration cells, we probed whether p68 and CaM would exhibit similar localization patterns. To this end, scratch-wounds were introduced to SW480 cells. The cells were then analysed by immunostaining. p68 and CaM clearly colocalized, especially at the leading edge of the migration cells. In the non-migrating cells, p68 localized exclusively in the nucleus, whereas CaM could be detected almost everywhere in the cells. However, there were significant increases in CaM levels at the leading edges and the nucleus in the migrating cells compared with that in non-migrating cells ( Fig. 3f ). We further examined the localizations of HA-p68 mutants LGLD and IQ-M and the effects of their expression on the cellular localization of CaM under scratch-wound conditions. Endogenous p68 was knocked down. The HA-p68s, WT, LGLD, or IQ-M was expressed in the cells. Scratch-wounds were subsequently introduced. Immunostaining using anti-HA antibody showed that WT HA-p68 localized to the leading edge of migrating cells. The ATPase-deficient mutant LGLD, although detected in the nucleus and the cytoplasm, failed to accumulate at the membrane edge. Interestingly, the IQ-M almost exclusively localized in the cell nucleus ( Fig. 3f ). Immunostaining of CaM in the same HA-p68s-expressing cells revealed that CaM also failed to accumulate at the membrane edge of the cells that expressed LGLD or IQ-M mutants under scratch-wound conditions ( Fig. 3f ). The results suggested that the p68–CaM interaction and the ATPase activity of p68 were required for the localization of CaM to the leading edge during cell migration. p68 exhibits CaM-dependent MT motor activity Redistribution of CaM to the leading edge areas is essential for cell migration [24] , [45] . However, the molecular mechanism governing the localization of CaM to the leading edge is not well understood. It is documented that MT motors are responsible for transportation of various molecules to the leading edge of migrating cells. We questioned whether p68 could mediate CaM and MT motor interactions in the migrating cells. Thus, we probed by coimmunoprecipitation interactions between p68 and two well-known MT motor molecules, kinesin and Dynein, in cell extracts prepared from SW480 cells that were treated by multiple scratch-wounds. No coprecipitations of either endogenous p68 or exogenous HA-p68 with the selected motor molecules were observed ( Supplementary Fig. S4a ). As the ATPase activity of p68 was required for CaM to localize to the leading edge of the migration cells, we considered whether p68 itself could have a role in translocation of CaM to the leading edge in migrating cells by acting as an unconventional MT-associated motor [17] , [18] . To test this conjecture, we first analysed whether p68 and/or CaM interact with MTs. p68/CaM and MT interactions were first analysed by MT coprecipitation assay. We carried out coprecipitation experiments with HA-p68 that was immunopurified from lysates of SW480 cells with/without multiple scratches ( Supplementary Fig. S4b ). The purified HA-p68 was incubated with MTs. After precipitation of the MTs by centrifugation, the presence of the HA-p68 in the MT precipitates was examined by immunoblot using an anti-HA antibody. HA-p68 that was purified from cells that were treated by scratch-wounds coprecipitated with MTs in the presence of CaM. In contrast, HA-p68 immunopurified from SW480 cells that were not treated by scratch-wounds did not coprecipitate with MTs even in the presence of CaM ( Fig. 4a ). The HA-p68 did not coprecipitate with unpolymerized α- and β-tubulin in the presence of Ca 2+ and CaM ( Supplementary Fig. S4c ). Interestingly, coprecipitation of HA-p68 with MTs in the presence of CaM was completely Ca 2+ dependent, whereas ATP was dispensable as the HA-p68 coprecipitated with the MT in the presence and absence of ATP, and in the presence of non-hydrolysable ATP analogue AMP-PNP ( Fig. 4b ). 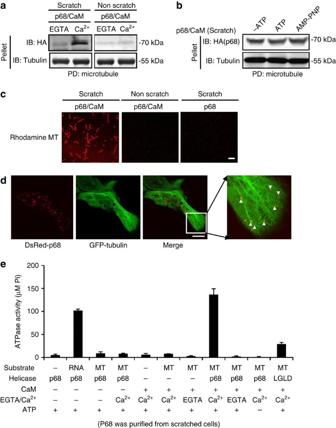Figure 4: p68 and CaM interact with microtubules. (a,b) Precipitation of HA-p68 that was immunopurified from cell lysates of multiple scratch-wound-treated (scratch) or untreated (non scratch) SW480 cells within vitroassembled microtubule (pellet) in the presence of CaM (p68/CaM) was probed by immunoblot of the precipitated pellets using the anti-HA antibody (IB:HA). The precipitations were carried out in the presence of 0.5 mM CaCl2(Ca2+) or 5 mM EGTA (EGTA) (a), or in the presence (ATP) and absence (−ATP) of ATP or in the presence of non-hydrolysable ATP analogue AMP-PNP (AMP-PNP) in addition to the presence of 0.5 mM CaCl2(b). Immunoblot analyses of α-tubulin (IB:Tubulin) is the loading control indicating amounts of precipitated microtubule. (c) Representative fluorescence microscopy images reveal the bindings of rhodamine-labelled microtubule (rhodamine MT) to the glass slides on which the HA-p68 that was immunopurified from cell lysates of multiple scratch-wound-treated (scratch) or untreated (non scratch) SW480 cells was attached (in the presence of CaM and Ca2+[p68/CaM] and absence of CaM [p68]). (d) Representative fluorescence microscopy images of SW480 cells that expressed DsRed-p68 and eGFP-α-tubulin. The cells were treated by scratch-wound. The arrows indicated the DsRed-p68. (e) ATPase activities of HA-p68 or mutant (indicated) that was immunopurified from cell lysates of multiple scratch-wound-treated SW480 cells in the presence of various different substrates (indicated) were analysed by measuring inorganic phosphate released from ATP hydrolysis. The ATPase activities were measured in the presence of 0.5 mM CaCl2(Ca2+) or 5 mM EGTA (EGTA), and in the presence and absence of the recombinant CaM. In the ATPase assays, 4 mM ATP was always added unless specified (-ATP). The ATPase activity was expressed as μmole of inorganic phosphate hydrolyzed from ATP. MT isin vitroassembled microtubule. RNA is total RNA extracts from yeast. Scale bars, 5 μm (forc) and 10 μm (ford). Figure 4: p68 and CaM interact with microtubules. ( a , b ) Precipitation of HA-p68 that was immunopurified from cell lysates of multiple scratch-wound-treated (scratch) or untreated (non scratch) SW480 cells with in vitro assembled microtubule (pellet) in the presence of CaM (p68/CaM) was probed by immunoblot of the precipitated pellets using the anti-HA antibody (IB:HA). The precipitations were carried out in the presence of 0.5 mM CaCl 2 (Ca 2+ ) or 5 mM EGTA (EGTA) ( a ), or in the presence (ATP) and absence (−ATP) of ATP or in the presence of non-hydrolysable ATP analogue AMP-PNP (AMP-PNP) in addition to the presence of 0.5 mM CaCl 2 ( b ). Immunoblot analyses of α-tubulin (IB:Tubulin) is the loading control indicating amounts of precipitated microtubule. ( c ) Representative fluorescence microscopy images reveal the bindings of rhodamine-labelled microtubule (rhodamine MT) to the glass slides on which the HA-p68 that was immunopurified from cell lysates of multiple scratch-wound-treated (scratch) or untreated (non scratch) SW480 cells was attached (in the presence of CaM and Ca 2+ [p68/CaM] and absence of CaM [p68]). ( d ) Representative fluorescence microscopy images of SW480 cells that expressed DsRed-p68 and eGFP-α-tubulin. The cells were treated by scratch-wound. The arrows indicated the DsRed-p68. ( e ) ATPase activities of HA-p68 or mutant (indicated) that was immunopurified from cell lysates of multiple scratch-wound-treated SW480 cells in the presence of various different substrates (indicated) were analysed by measuring inorganic phosphate released from ATP hydrolysis. The ATPase activities were measured in the presence of 0.5 mM CaCl 2 (Ca 2+ ) or 5 mM EGTA (EGTA), and in the presence and absence of the recombinant CaM. In the ATPase assays, 4 mM ATP was always added unless specified (-ATP). The ATPase activity was expressed as μmole of inorganic phosphate hydrolyzed from ATP. MT is in vitro assembled microtubule. RNA is total RNA extracts from yeast. Scale bars, 5 μm (for c ) and 10 μm (for d ). Full size image The interaction of p68–CaM with MTs was further examined by binding of rhodamine-labelled MTs to HA-p68 that was fixed on a glass slide. Binding of the MT to the glass slide was then visualized by fluorescence microscopy. The MTs clearly bound to the HA-p68 purified from scratch-wound-treated SW480 cells in the presence of CaM and Ca 2+ . The MTs did not bind HA-p68 without addition of CaM ( Fig. 4c ). The MTs also did not bind to HA-p68 that was purified from SW480 cells that were not treated by scratch-wounds ( Fig. 4c ). We further examined the colocalization of DsRed-p68 with MTs labelled by eGFP. Under scratch-wound treatment, DsRed-p68 clearly colocalized with eGFP-labelled MTs ( Fig. 4d ). Thus, we could draw the conclusion that p68 interacts with MTs and the interaction is dependent upon p68–CaM interaction. If p68 could function as a MT motor-like molecule, we would expect that MTs would stimulate ATPase activity of p68. Thus, the ATPase activity of the HA-p68 that was immunopurified from SW480 cells ( Supplementary Fig. S4b ) treated with multiple scratch-wounds was analysed in the presence of various different possible substrates, including RNA and MTs. As previously reported [46] , HA-p68 exhibited strong RNA-dependent ATPase activity. Interestingly, the protein demonstrated an even stronger MT-stimulated ATPase activity ( Fig. 4e ), and the MT-stimulated ATPase activity was Ca 2+ dependent as addition of EGTA diminished it ( Fig. 4e ). The observed MT-stimulated ATPase activity came from p68 as the mutation that abolishes p68 ATPase activity (LGLD) also abolished the MT-stimulated ATPase activity of the protein ( Fig. 4e ). In addition, this MT-dependent ATPase activity was not detected with the HA-p68 purified from the cells extracts without scratches ( Supplementary Fig. S4d ). We next probed whether p68 indeed has MT motor activity. To this end, we employed MT gliding assays. HA-p68 was purified from SW480 cells with scratches and attached to a glass slide. Rhodamine-labelled MTs were then added to the glass slide. Migration of the MT in the presence and absence of ATP was then recorded. First, migration of MTs was clearly visualized with a positive control motor protein kinesin ( Fig. 5a , Supplementary Movie 1 ). Migration of the MTs on the glass slide with HA-p68 attached was also clearly evident in the presence of CaM and Ca 2+ . As a negative control, migration was not observed without addition of ATP ( Fig. 5a , Supplementary Movie 2 ). Statistical analyses indicated that the HA-p68/CaM complex exhibits motor activity on MTs very similar to that of a control motor kinesin (the number of gliding microtubles, mean gliding speed and maximum gliding speed in a random selected group of 50 are similar, Table 1 ). As p68 and HA-p68 did not coimmunoprecipitate with two very common MT-associated motor proteins ( Fig. 5b ), it is less likely that the observed HA-p68 motor activity is due to copurification of residual other cellular motor proteins. To further exclude the possibility that the motor activity was due to contamination during purification, we constructed a p68–CaM fusion protein ( Supplementary Fig. S5a ). On the basis of computational modelling ( Supplementary Fig. S6 ), the C-terminus of p68 is a flexible loop and is located close to the IQ-like motif. Thus, the fusion should bring the CaM in proximity to the IQ-like motif. Expression of the HA-p68–CaM fusion protein in SW480 cells led to greatly increased cell migration ( Supplementary Fig S5b,c ) and the expressed fusion protein localized to the leading edge of migrating cells. In fact, expression of the fusion protein promoted formation of lamellipodia/filopodia without scratch-wounding ( Supplementary Fig S5d ). These observations indicated that the fusion protein functionally resembles the p68–CaM complex induced by migration signals. We then expressed and purified the fusion protein His-p68–CaM from E. coli . Gliding assays was performed with this bacterially expressed fusion protein. The bacterially expressed His-p68–CaM binds to MTs ( Supplementary Fig. S5e ), possesses MT-dependent ATPase activity ( Supplementary Fig. S5f ), and has strong MT motor activity ( Fig. 5a and Table 1 ). 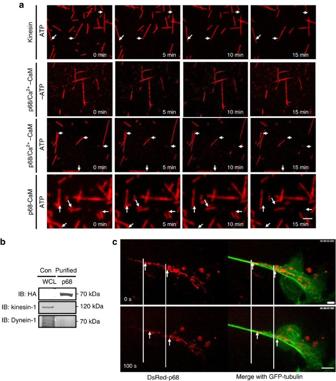Figure 5: p68–CaM has microtubule motor activity. (a) The movements of rhodamine-labelled microtubules on the glass slides on which the immunopurified HA-p68 (from SW480 cells) or bacterially expressed His-p68–CaM (p68–CaM) was attached in the presence (ATP) and absence (−ATP), and in the presence of 0.5 mM CaCl2were recorded by the time lapse photography with confocal fluorescence microscopy (seeSupplementary Movies 1and2). (b) Existence of Kinesin-1 and Dynein-1 in the HA-p68 immunopurification was analysed by immunoblots of the purified HA-p68 (IB:HA) using antibodies against kinesin-1 (IB:kinesin-1) and Dynein-1 (IB:Dynein-1). (c) Movements of DsRed-p68 along eGFP-labelled microtubules in SW480 cells that were treated by scratch-wound were recorded by time lapse photography with confocal fluorescence microscopy (seeSupplementary Movie 3). Ina, arrows indicate the same positions of different time points. Inc, the arrows indicate the moved DsRed-p68. Scale bar, 5 μm (foraandc). Figure 5: p68–CaM has microtubule motor activity. ( a ) The movements of rhodamine-labelled microtubules on the glass slides on which the immunopurified HA-p68 (from SW480 cells) or bacterially expressed His-p68–CaM (p68–CaM) was attached in the presence (ATP) and absence (−ATP), and in the presence of 0.5 mM CaCl 2 were recorded by the time lapse photography with confocal fluorescence microscopy (see Supplementary Movies 1 and 2 ). ( b ) Existence of Kinesin-1 and Dynein-1 in the HA-p68 immunopurification was analysed by immunoblots of the purified HA-p68 (IB:HA) using antibodies against kinesin-1 (IB:kinesin-1) and Dynein-1 (IB:Dynein-1). ( c ) Movements of DsRed-p68 along eGFP-labelled microtubules in SW480 cells that were treated by scratch-wound were recorded by time lapse photography with confocal fluorescence microscopy (see Supplementary Movie 3 ). In a , arrows indicate the same positions of different time points. In c , the arrows indicate the moved DsRed-p68. Scale bar, 5 μm (for a and c ). Full size image Table 1 Motor activity of p68/CaM and p68–CaM fusion. Full size table Finally, we examined whether p68 indeed migrates along MTs in cells that are induced to migrate. p68 fused with DsRed (DsRed-p68) and eGFP-labelled α-tubulin were coexpressed in SW480 cells. Cell migration was induced by scratch-wounds. Movement of the DsRed-p68 along the eGFP-labelled MT was recorded using confocal microscope with multi-photon excitation for imaging of living cells with time lapse photography. The fluorescence images clearly indicated that DsRed-p68 migrated along the MT under cell migration induction. The movements were towards the migration leading edge ( Fig. 5c , Supplementary Movie 3 ). The results suggest that by interacting with CaM, p68 RNA helicase can function as a MT motor. PepIQ inhibits metastasis in a 4T1 orthotopic model PepIQ was very effective in inhibiting cancer metastasis in a xenograft model using SW620 cells, suggesting a potential application for metastasis intervention using the peptide or its derivatives. Thus, we tested the effects of the peptide on inhibition of cancer metastasis in another cancer model. Mouse breast cancer 4T1 cells were implanted into the mammary glands of Balb/c mouse. Four days post tumour implantation, the mice were treated with buffer alone or with PepIQ or the control peptide (PepScram) at a 2 mg kg −1 daily dose for 14 days via intraperitoneal (i.p.) injection. The mice were killed 26 days after tumour implantation. The primary tumours and major metastasis organs (lungs and liver) were collected and examined. It was evident that the peptide treatments did not lead to any significant change in primary tumour growth ( Fig. 6a , a tumour in one mouse in the PepIQ-treated group did not grow). Strong metastasis to the lung with multiple metastasis sites was observed in the buffer and the PepScram treatment groups, whereas only three out of four mice displayed lung metastases in the PepIQ-treated group (one mouse was completely metastasis free in the lungs). The numbers of visible metastatic nodules in the lungs of the PepIQ-treated group were much less and the nodules were much smaller than those in the PepScram and buffer-treated groups ( Fig. 6b–d ). No visible metastasis nodules were observed in livers of all mice. However, histological analyses revealed micrometastasis lesions in the livers ( Fig. 6e ). Quantification of the micrometastasis lesions in four randomly selected fields from three randomly selected tissue sections of the liver from each mouse revealed that the average numbers of micrometastasis lesions were substantially less in the PepIQ-treated group compared with those of buffer and PepScram-treated groups ( Fig. 6f ). No micrometatstasis lesions were seen in the liver tissue sections from two out of four mice in the PepIQ-treated group. The size of micrometastasis lesions in the PepIQ-treated group was also substantially smaller than that of control groups (data not shown, and see Fig. 6e ). To test whether PepIQ also affected the migration of 4T1 cells, we carried out cell migration assays. Both Boyden chamber and scratch-wound assays indicated that cell migration was dramatically reduced upon the PepIQ treatment ( Supplementary Fig. S6a ,b). 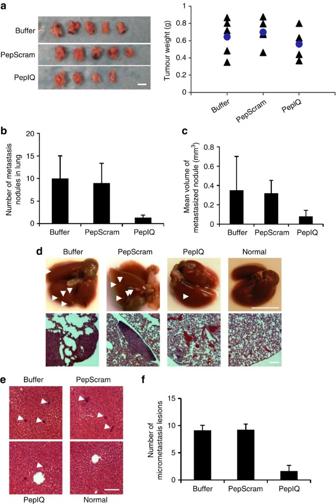Figure 6: PepIQ inhibits metatstasis of 4T1 tumours. (a) Pictures (left) and weight (right) of harvested 4T1 tumours after 26 days growth with 14 days treatment using the indicated peptides. (b,c) The numbers (b) and sizes (c) of the metastasis nodules in the lung of 4T1 tumour-bearing mice that were treated by different peptides (indicated) by physical inspection. (d, upper) representative lungs collected from 4T1 tumour-bearing mice that were treated by different peptides (indicated). Arrows indicate the metastasis nodules. (d, bottom) Representative images of H&E staining of tissue sections of lungs from 4T1 tumour-bearing mice that were treated by different peptides (indicated). (e) Representative images of H&E staining of tissue sections of livers from 4T1 tumour-bearing mice that were treated by different peptides (indicated). Arrows indicate micrometastasis lesions. (f) The numbers of the micrometastasis lesions in the tissue sections of liver of 4T1 tumour-bearing mice that were treated by different peptides (indicated). The numbers of micrometastasis lesion were counted by randomly selected four fields from randomly selected three tissue sections of each liver. TheP-values (between ‘pepscram’ and ‘pepIQ’,P=0.297525 ina, between ‘pepscram’ and ‘pepIQ’,P=0.005257 inb, between ‘pepscram’ and ‘pepIQ’,P=0.038065 incand between ‘pepscram’ and ‘pepIQ’,P=1.71745E−08inf) are calculated by the pairwise Student’st-tests. Scale bars, 1 cm (foraandd(upper panel)) and 200 μm (ford(lower panel) ande). Figure 6: PepIQ inhibits metatstasis of 4T1 tumours. ( a ) Pictures (left) and weight (right) of harvested 4T1 tumours after 26 days growth with 14 days treatment using the indicated peptides. ( b , c ) The numbers ( b ) and sizes ( c ) of the metastasis nodules in the lung of 4T1 tumour-bearing mice that were treated by different peptides (indicated) by physical inspection. ( d , upper) representative lungs collected from 4T1 tumour-bearing mice that were treated by different peptides (indicated). Arrows indicate the metastasis nodules. ( d , bottom) Representative images of H&E staining of tissue sections of lungs from 4T1 tumour-bearing mice that were treated by different peptides (indicated). ( e ) Representative images of H&E staining of tissue sections of livers from 4T1 tumour-bearing mice that were treated by different peptides (indicated). Arrows indicate micrometastasis lesions. ( f ) The numbers of the micrometastasis lesions in the tissue sections of liver of 4T1 tumour-bearing mice that were treated by different peptides (indicated). The numbers of micrometastasis lesion were counted by randomly selected four fields from randomly selected three tissue sections of each liver. The P -values (between ‘pepscram’ and ‘pepIQ’, P =0.297525 in a , between ‘pepscram’ and ‘pepIQ’, P =0.005257 in b , between ‘pepscram’ and ‘pepIQ’, P =0.038065 in c and between ‘pepscram’ and ‘pepIQ’, P =1.71745E −08 in f ) are calculated by the pairwise Student’s t -tests. Scale bars, 1 cm (for a and d (upper panel)) and 200 μm (for d (lower panel) and e ). Full size image We present evidence to demonstrate that strengthening the interaction of p68 with CaM is required for cell migration. Disrupting the p68–CaM interaction effectively inhibits cancer metastasis in two different animal models, suggesting a potential new approach for metastasis intervention. The actions of the PepIQ in inhibiting cancer metastasis provide a proof-of-principle that the strategy of disrupting the p68–CaM interaction can be a target for the development of antimetastasis agents. Using the peptide may not be ideal pharmacologically. However, study with the peptide certainly provides important guidance for the further design of new molecules that can disrupt p68–CaM interaction and stop cancer metastasis. p68 was shown to interact with CaM by several independent in vitro analyses [36] , [37] , [38] . However, the actual interaction site(s) is not certain. The IQ region of p68 does not match a complete consensus sequence of IQ motif, rather an incomplete IQ-like motif characterized by (FILV)Qxxx(RK)xxxxx. The x represents any amino acid. Studies show that the IQ-like motif binds to CaM with various affinities [47] , [48] . The biological function of p68–CaM interaction is not known. Our results suggested that the p68–CaM interaction is necessary for localization of CaM to the migration leading edge, which is an essential event during cell migration. p68, by interacting with CaM, exhibited a MT motor activity. Apparently, this motor activity allows CaM to be transported to the leading edge of migrating cells. On the basis of our current findings, our working model for the role of p68 in cell migration is illustrated in Fig. 7 . Interestingly, p68 stays at the leading edge of migrating cells until the cell reaches its migration destination, indicating possible additional function(s) of p68 at the migration leading edge during migration. One possibility is that p68 may also have a role in leading edge protrusion, for example, actin filament polymerization. 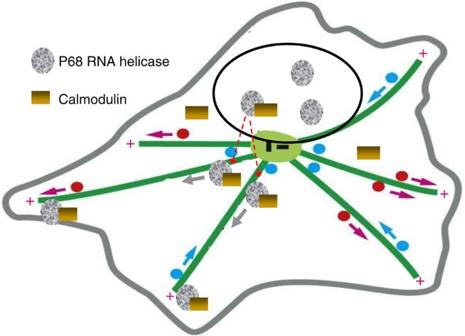Figure 7: Model of p68–calmodulin function in cell migration. A hypothetical model that illustrates the functions of p68 and CaM interaction in cell migration, and the microtubule motor actions of p68 upon interacting with CaM. Figure 7: Model of p68–calmodulin function in cell migration. A hypothetical model that illustrates the functions of p68 and CaM interaction in cell migration, and the microtubule motor actions of p68 upon interacting with CaM. Full size image CaM regulates various cellular processes by targeting over a hundred proteins. A key feature for such functional diversity is temporal and spatial redistribution of the protein under stimulation by various different signalling pathways [24] , [25] . A long-standing question is how CaM is translocated to a specific subcellular compartments. We demonstrated an excellent example here, in which p68 interacts with CaM upon cell migration stimulation. This interaction allows p68 to interact with MTs and to subsequently act as a MT motor, which consequently transports the bound CaM to the leading edge of migrating cells. An open question is whether a similar mechanism is also used to relocalize CaM in other cellular processes that require temporal and spatial redistribution of CaM, such as cytokinesis and mitosis. It is traditionally believed that DEAD box RNA helicases use RNA as a substrate to stimulate ATPase activity. The energy is then used to displace duplex RNA or proteins that bind the RNA substrate. Along with our previously published observations [31] , this is the second example showing that p68 RNA helicase can use protein as a substrate to stimulate its ATPase activity. It is conceivable that the energy derived from ATP hydrolysis can be used for translocation along the MT (motor-like protein). However, a typical MT motor binds MTs with two ‘motor head’. The movement along the MT is usually driven by cyclic hydrolysis of ATP at the two heads [49] . Thus, an open question is how the p68 motor action on MTs is achieved by one ATP hydrolysis site. One possibility is that the bound CaM may function as an anchor, while ATP hydrolysis in p68 powers the movement. This scenario would require that CaM interact with MTs. Nevertheless, the interaction between CaM and MT is not observed. Alternatively, p68 RNA helicase may travel along the MT using a mechanism similar to that used by a DEAD box RNA helicase translocating along an RNA substrate [50] . Experimental materials The HA peptide was synthesized by AnaSpec. Polyclonal (Pabp68) and monoclonal (p68-RGG) antibodies against p68 were the same as previously reported [32] . Antibodies HA-tag, GAPDH, Lamin A/C, CaM, α-tubulin, β-tubulin, heavy chain of kinesin-1, Dynein intermediate 1 and β-actin were purchased from Cell Signaling, Abnova, SantaCruz, Abcam and AnaSpec, respectively. Microtubule and rodamine-labelled MT were purchased from Cytoskeleton. Cell line SW480/SW620 and 4T1 were purchased from ATCC and cultured by following the vendor’s instructions. HA-tagged p68 encoding DNA sequence was cloned into the pHM6 vector. Calmodulin beads pull-down Whole-cell lysate from SW480 cells was prepared according to the procedure described in our previous report [31] , [32] . The agarose beads conjugated with recombinant calmodulin (Abcam) were prewashed with Ca 2+ containing buffer (2 mM CaCl 2 , 50 mM NaCl in 50 mM Tris–HCl pH7.5) or EGTA containing buffer (5 mM EGTA, 50 NaCl in 50 mM Tris–HCl pH7.5). After washing, the beads were incubated with the whole-cell lysates in the Ca 2+ containing or EGTA containing buffer. The beads were extensively washed after incubation. Finally, 2 × SDS-loading buffer were added to the beads and the beads were heated to 85 °C for 10 min. The proteins that were pulled down by the CaM beads were analysed by 10% SDS–polyacrylamide gel electrophoresis (SDS–PAGE) and subsequent immunoblot. Boyden chamber assay QCM 24-Well Fluorimetric Cell Migration Assay kit (ECM) was used to measure the migration of SW480 cells. The test cells were first treated under the different conditions (indicated in figure legends) in regular cell culture plates. The treated cells were resuspended into optimum medium (without serum) and seeded into the inner chamber of the migration assay kit. The L-15 culture medium with 10% fetal bovine serum was added to the outer chambers. After overnight incubation, medium in the inner chamber was removed and the cells attached to the outer bottom side were detached using the cell-detachment buffer (included in the kit). The detached cells were then lysed using the cell lysis buffer (included in the kit). The amounts of the migrated cells were determined by measuring the fluorescence using λ ex=485 nm and λ em=535 nm. The migration of the control cells with p68 knockdown was defined as 1. Immunopurification of HA-tagged proteins from cell extracts SW480 cells expressing HA-tagged proteins by transient transfection were cultured in medium L-15 with 10% fetal bovine serum. The cells were subjected to different treatment (such as scratch-wounds). The cells were collected and lysed in NETS buffer with addition of the protease inhibitors. To minimize the non-specific protein–protein interactions in the immunopurification, 600 mM (final concentration) 6-aminocaproic acid along with 800 mM (final concentration) NaCl were added to the extracts and incubated for 2 h at room temperature (RT). A commercially available polyclonal anti-HA antibody was added to the prepared extracts (500 μl extracts per 20 μl of Abs). The mixture was incubated overnight at 4 °C. After incubation, the protein G agarose beads (50 μl, pretreated with bovine serum albumin (BSA; 3 mg ml −1 ) were then added to the mixture and incubated for an additional 2 h. The beads were washed in NETS buffer six times. The beads bound proteins were either directly used in some assays (such as ATPase assays) or the bound HA-tagged proteins were eluted using the HA peptide. The beads with bound proteins were suspended in elution buffer and packed in a small column. The HA peptide (Sigma) (500 μg ml −1 in elution buffer) was flowed through the column to elute the bead-bound proteins. The fractions were collected and analysed by SDS–PAGE and immunoblot to identify the fractions that contained HA-tagged protein. The eluted proteins were further dialyzed in the subsequent assay buffers (such as MT binding buffer) and concentrated by centrifugation. ATPase assays The ATPase activity of different proteins (specified in figures and legends) was assayed by an experimental procedure similar to that described previously with minor modifications [44] , [46] . The reaction volume was 50 μl, containing 4 μg of MTs (or 2 μg of RNA), 4 mM ATP and 0.5 mM Ca 2+ or 5 mM EGTA in the ATPase assay buffer (10 mM Pipes pH 7.0, 1 mM MgCl 2 , 25 mM NaCl with taxol added). Ten microlitres of the purified HA-tagged proteins (bound or unbound to agarose beads) was added. The ATPase reactions were incubated for 30 min at 37 °C. After incubation, 30 μl of the supernatant was added to 1 ml of malachite green-molybdenum reagent. After 5 min incubation at RT, the absorbance of the reaction was then measured at 630 nm (A630). The concentrations of released inorganic phosphate were determined by matching the A630 nm in a standard curve of A630 nm versus known phosphate concentrations. Metastasis inhibition of xenograft tumours All animal experiments were carried out in accordance with the guidelines of IACUC of Georgia State University. Nude mice or Balb/c mice (6–7 weeks old, Harlan Laboratory) were subcutaneously or orthotopically injected with 5 × 10 6 SW620 or 2 × 10 6 4T1 cells. Peptides at appropriate doses were i.p. injected to the tumour-bearing mice at appropriate time intervals. Tumour formation and volumes were assessed every 3 days. Tumour volumes were measured by two perpendicular diameters of the tumours over a 4-week time course with the formula 4p/3 × (width/2) 2 × (length/2). The tumours and organs were collected and weighed at the end of the experiments. Tissue sections were prepared from harvested tumours and organs. Tissue sections were analysed by either haematoxylin and eosin (H&E) or immune fluorescence staining. For metastasis analyses of SW620 tumours, tissue extracts were prepared from spleens, total RNAs were extracted from the tissue extracts. RT–PCRs were performed with the isolated RNAs. For metastasis of 4T1 cells, lung and liver were inspected. Tissue sections were also prepared and analysed by H&E or immune staining. Statistical analyses were done in comparison with the control group with a paired Student’s t- test. Scratch-wound treatments A scratch or multiple scratches using pipette tips were introduced into a six-well cell culture plate. The cells were further cultured under serum starvation for 30 min, and were subsequently cultured for an additional indicated time. The scratch-treated cells were either directly visualized by microscopes or the cells were fixed and subsequently examined by immunostaining. Alternatively, the cells were collected and lysized. The prepared cellular extracts were then used for other analyses. Microtubule pull-down and gliding assay Microtubule purchased was reconstituted in warm PM buffer (15 mM Pipes pH 7.0, 1 mM MgCl 2 ) with the addition of taxol as instructed by the vendor. The MTs were ready to use after 15-min incubation at RT. The test protein(s) was incubated with the reconstituted MTs under various conditions. The MTs with the bound proteins were separated from the incubation solution by centrifugation at 100,000 g for 30 min. Coprecipitates with the MTs were resuspended in 50 μl of 2 × SDS–PAGE loading buffer and heated to 85 °C for 10 min and subsequently analysed by immunoblots. The protein HA-p68–CaM, HA-p68 or His-p68–CaM (10 μl) (pretreated by RNase cocktail, RNase A, T1 and V1) was loaded onto a glass slide. The slide was blocked with the blocking buffer. For the slide loaded with HA-p68, 10 μl of calmodulin with 0.5 mM of Ca 2+ was added to the slide and was incubated for 10 min. After loading the slide was washed with the Ca 2+ containing wash buffer to remove the unbound proteins. The prepared rodamine-labelled MTs were then loaded onto the slide. The same Ca 2+ containing wash buffer was used to remove unbound MTs. The movement of MTs was then recorded by the confocal microscope. How to cite this article: Wang, H. et al . Interaction between p68 RNA helicase and Ca 2+ -calmodulin promotes cell migration and metastasis. Nat. Commun. 4:1354 doi: 10.1038/ncomms2345 (2013).